Emergence of electric-field-tunable interfacial ferromagnetism in 2D antiferromagnet heterostructures Van der Waals (vdW) magnet heterostructures have emerged as new platforms to explore exotic magnetic orders and quantum phenomena. Here, we study heterostructures of layered antiferromagnets, CrI 3 and CrCl 3 , with perpendicular and in-plane magnetic anisotropy, respectively. Using magneto-optical Kerr effect microscopy, we demonstrate out-of-plane magnetic order in the CrCl 3 layer proximal to CrI 3 , with ferromagnetic interfacial coupling between the two. Such an interlayer exchange field leads to higher critical temperature than that of either CrI 3 or CrCl 3 alone. We further demonstrate significant electric-field control of the coercivity, attributed to the naturally broken structural inversion symmetry of the heterostructure allowing unprecedented direct coupling between electric field and interfacial magnetism. These findings illustrate the opportunity to explore exotic magnetic phases and engineer spintronic devices in vdW heterostructures. Heterostructures are promising to host emergent phenomena and device functions not present in constituent parts [1] , [2] , [3] , [4] , [5] , [6] , [7] , [8] , [9] , [10] . One well-known example is the integration of two insulating complex oxides leading to a conducting two-dimensional electron gas at the interface [2] , with surprising coexistence of superconductivity and ferromagnetism [3] . The recently explored van der Waals (vdW) magnets have pushed the research frontier to 2D magnetism where exotic magnetic ground states and quantum phases can emerge [11] , [12] , [13] , [14] , [15] , [16] , [17] , [18] . Magnetic vdW heterostructures provide a new toolbox to explore magnetic proximity and related effects [4] , [5] , [6] , [7] , [8] , [9] , [10] . A largely unexplored arena is to combine two different magnetic orders and investigate the magnetic proximity at the interface, which could allow modulation of magnetic interactions and establish exotic magnetic properties. It is also of fundamental significance to effectively control the exchange interactions and magnetic anisotropy, with the latter being crucial to stabilize the long-range magnetic orders. The studies of layered semiconducting chromium trihalides have shown exotic magnetic behaviors and rich tunability by stimuli [14] , [15] , [16] , [17] , [18] . Typically, the few-layer (FL) CrI 3 is an antiferromagnet with Ising-like perpendicular magnetic anisotropy (PMA) [19] , [20] , as schematically depicted in Fig. 1a . The interlayer antiferromagnetic coupling is ascribed to the exchange interactions between Cr mediated by ligand atoms [17] , [20] . In contrast, FL CrCl 3 is an easy-plane interlayer antiferromagnet, where spins prefer to lie in the layers [20] , [21] . In particular, the single-ion anisotropy from spin-orbit coupling (SOC) of Cr and the anisotropic exchange from SOC of Cl nearly cancel out each other [20] , [21] . Therefore, CrCl 3 is located close to the boundary between PMA and in-plane anisotropy, suggesting that its magnetic properties may be particularly susceptible to external perturbations. The combined heterostructure of CrI 3 and CrCl 3 is possibly a fertile system to realize rich magnetic phases and manipulate them. Such a heterostructure has not yet been explored. Fig. 1: CrI 3 /CrCl 3 heterostructures and MOKE measurements. a Schematics of the magnetic ground states in bilayer (2L) CrI 3 and few-layer (FL) CrCl 3 before (left) and after (right) forming heterostructure. Only four layers of CrCl 3 are shown for simplicity. b Optical micrograph of a 2L CrI 3 /FL CrCl 3 heterostructure. c Atomic force microscopy of the heterostructure in the same position as in b . The height profile (along the yellow dotted line in the image) at the edge of CrI 3 indicates the thickness of a bilayer. d MOKE signal (after subtracting a polynomial background, as done for all MOKE curves in the main text) of the 2L CrI 3 region and the 2L CrI 3 /FL CrCl 3 heterostructure region as a function of perpendicular magnetic field. Two curves of each region represent forward and backward sweeps of the field, respectively. The data are taken at the spots marked by red in b . Insets depict magnetic ground states of 2L CrI 3 and the CrI 3 /CrCl 3 heterostructure (showing only the interfacial CrCl 3 layer, highlighted by red dashed rectangles). e MOKE signal of another monolayer (1L) CrI 3 /FL CrCl 3 heterostructure, compared with that measured in the 1L CrI 3 (from the same CrI 3 flake as in the heterostructure region). Full size image Here, we fabricate CrI 3 /CrCl 3 heterostructures and demonstrate interfacial ferromagnetism between the two antiferromagnets. 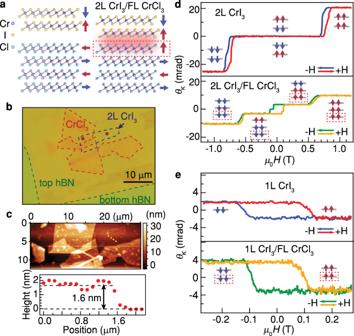Fig. 1: CrI3/CrCl3heterostructures and MOKE measurements. aSchematics of the magnetic ground states in bilayer (2L) CrI3and few-layer (FL) CrCl3before (left) and after (right) forming heterostructure. Only four layers of CrCl3are shown for simplicity.bOptical micrograph of a 2L CrI3/FL CrCl3heterostructure.cAtomic force microscopy of the heterostructure in the same position as inb. The height profile (along the yellow dotted line in the image) at the edge of CrI3indicates the thickness of a bilayer.dMOKE signal (after subtracting a polynomial background, as done for all MOKE curves in the main text) of the 2L CrI3region and the 2L CrI3/FL CrCl3heterostructure region as a function of perpendicular magnetic field. Two curves of each region represent forward and backward sweeps of the field, respectively. The data are taken at the spots marked by red inb. Insets depict magnetic ground states of 2L CrI3and the CrI3/CrCl3heterostructure (showing only the interfacial CrCl3layer, highlighted by red dashed rectangles).eMOKE signal of another monolayer (1L) CrI3/FL CrCl3heterostructure, compared with that measured in the 1L CrI3(from the same CrI3flake as in the heterostructure region). Figure 1a left panel schematically depicts the expected spin configurations for the magnetic ground states in bilayer (2L) CrI 3 and FL CrCl 3 with PMA and in-plane anisotropy [19] , [20] , [21] , respectively. Due to the strong intralayer ferromagnetic coupling in chromium trihalides [17] , we can denote all spins in a given layer by a macroscopic spin (out-of-plane: ↑, ↓; in-plane: ←, →). The optical micrograph of a representative 2L CrI 3 /FL CrCl 3 heterostructure is shown in Fig. 1b . The 2L CrI 3 is partially stacked on top of FL CrCl 3 , allowing the comparison between regions of 2L CrI 3 , FL CrCl 3 and heterostructure. Atomic force microscopy (AFM) confirms flake thickness of 1.6 nm for 2L CrI 3 (Fig. 1c ) and 9.5 nm for FL CrCl 3 , respectively. We employ magneto-optical Kerr effect microscopy (MOKE) under the polar configuration as the primary measurement due to its high sensitivity to the magnetic moments perpendicular to the sample surface [22] . Figure 1d shows the MOKE signal ( θ K ) of the 2L CrI 3 and the 2L CrI 3 /FL CrCl 3 heterostructure as a function of the perpendicular magnetic field. In the 2L CrI 3 region, θ K stays close to zero at low field, corresponding to the antiferromagnetic states ↓ ↑ or ↑↓ with zero net magnetization. Beyond critical field ±0.76 T, θ K abruptly jumps to ferromagnetic states with finite magnetization. This is consistent with the reported spin-flip transitions in 2L CrI 3 [23] . In the 2L CrI 3 /FL CrCl 3 heterostructure, the antiferromagnetic-to-ferromagnetic spin-flip transition of 2L CrI 3 is still present and its critical field decreases from ±0.76 T in 2L CrI 3 region to ±0.57 T in the heterostructure region. Remarkably, a significant square hysteresis loop is observed with coercive field ~±0.1 T, indicating a magnetic transition between two different phases with non-zero net magnetization, in sharp contrast to the antiferromagnetic ground states in 2L CrI 3 (↓↑ or ↑↓). Such a ferromagnetic-like loop is absent in either 2L CrI 3 or FL CrCl 3 , suggesting its origin from interfacial magnetic interaction. This phenomenon should not be due to the charge transfer/doping-induced antiferromagnetic-to-ferromagnetic transition reported in 2L CrI 3 [14] , [15] , which does not exhibit such a coexistence of antiferromagnetic-type and ferromagnetic-type transitions. Recent works have shown that a twist of two chromium trihalides layers may lead to noncollinear antiferromagnetic-ferromagnetic domains and thus finite MOKE signals [9] , [10] , [18] , [24] , [25] , [26] , [27] . However, this scenario is also less likely to be relevant, as such domains are predicted to emerge for sufficiently large moiré periodicity. Due to large lattice constant mismatch [18] , the CrI 3 /CrCl 3 heterostructure can hardly form large moiré periodicity even at zero twist angle. Furthermore, the magnetization behaviors (including the field and temperature dependence) measured in twisted CrI 3 [9] , [10] , [25] , [26] , [27] exhibit qualitative difference from what we observe in our samples. We further rule out several other possible origins (see detailed discussions in Supplementary Text 1 ). We propose that at least three spin layers (two layers of CrI 3 plus one neighboring layer of CrCl 3 ) are responsible for the observed transitions. The neighboring CrCl 3 layer is acting as the third spin layer with out-of-plane magnetic order after being stacked in proximity with CrI 3 , as schematically shown in Fig. 1a and denoted in the red dashed rectangles in Fig. 1d, e . Note that a perpendicular magnetic field induces canting of the planar CrCl 3 spins, giving rise to a continuously varying MOKE background [28] (Supplementary Fig. 1 ), which is typically subtracted and eliminated from our MOKE signal. Therefore, only perpendicular spin-flip transitions are discussed in this work. Similar to trilayer CrI 3 , in principle several potential antiferromagnetic configurations can be considered: ↑↓↓ (−1), ↓↑↑ (+1), ↓↑↓ (−1), ↑↓↑ (+1) with the first two and the third spins referring to the 2L CrI 3 and the neighboring CrCl 3 layer respectively and the numbers in brackets denoting the net magnetic moments. To figure out the coupling type for the neighboring CrI 3 and CrCl 3 layers, we study the 1L CrI 3 /FL CrCl 3 heterostructure where the magnetic behavior can directly verify the interlayer coupling type. Figure 1e shows θ K of the 1L CrI 3 and the 1L CrI 3 /FL CrCl 3 heterostructure, fabricated from the same CrI 3 flake. Interestingly, both show a ferromagnetic behavior with a single hysteresis loop. This observation indicates that the neighboring CrI 3 and CrCl 3 layer is ferromagnetically coupled, in contrast to the interlayer antiferromagnetic coupling in FL CrI 3 [19] . Careful inspection on the hysteresis loop in Fig. 1d shows more transition steps, possibly due to the switching of magnetic domains [23] , [29] . Note that due to thin-film optical interference effect [23] , [30] . it is not possible to associate the magnitude or sign of the MOKE signal to the magnetization of different samples (e.g., the doubling of the MOKE signal in the 1L CrI 3 /FL CrCl 3 heterostructure relative to that in the 1L CrI 3 in Fig. 1e does not imply that the probed magnetization doubles). In the following text, we mainly focus on other features (e.g., emergent hysteresis loop, transition/coercive fields, critical temperatures). To exclude any unique causes related to the stacking sequence, we also studied reversely stacked heterostructures with FL CrCl 3 on top of 2L CrI 3 and observed similar hysteresis loops (Supplementary Figs. 2 and 3 ). The larger coercive field of the hysteresis loop observed in the reversed stack may be due to sample differences or twist angle dependence and is out of the scope of this work. We next study the temperature dependence of the magnetism in the heterostructure. 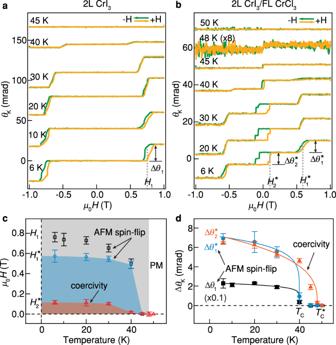Fig. 2: Temperature dependence of the magnetism of 2L CrI3and 2L CrI3/FL CrCl3heterostructure. MOKE signal in the 2L CrI3region (a) and the 2L CrI3/FL CrCl3heterostructure region (b) as a function of perpendicular magnetic field at different temperatures. Critical fieldsH1,H1*,H2*and magnitudes in the change of MOKE signal ∆θ1, ∆θ1*, ∆θ2*of magnetic transitions are labeled.cTemperature dependence of the critical fields of magnetic transitions. PM paramagnetic. The critical fields are extracted from the peak of derivative dθK/dHand the error bars are the peak widths.dTemperature dependence of the magnitudes in the change of MOKE signal at magnetic transitions. Solid curves are fitted by a power-law equation11. The critical temperaturesTCandTC*are indicated. The error bars are the uncertainties in extracting the transition magnitudes. Figure 2a, b shows the temperature dependence of θ K in 2L CrI 3 and 2L CrI 3 /FL CrCl 3 heterostructure. The extracted H 1 , H 1 * , H 2 * and ∆ θ 1 , ∆ θ 1 * , ∆ θ 2 * as a function of temperature are shown in Fig. 2c, d , respectively. The antiferromagnetic spin-flip transitions (at H 1 and H 1 * ) in both 2L CrI 3 and the heterostructure disappear at temperatures larger than T C ~ 40 K and is consistent with previous measurements in 2L CrI 3 [31] . The ferromagnetic-like hysteresis loop (at H 2 * ) observed only in the heterostructure region survives up to a higher temperature T C * ~ 48 K. Another experiment on 1L CrI 3 /FL CrCl 3 heterostructure shows critical temperatures of T C ~ 33 K and T C * ~ 37 K for 1L CrI 3 region and heterostructure region, respectively (Supplementary Fig. 4 ). In 2D magnets, the critical temperature is determined by the spin-wave excitation gap, which is dictated by the anisotropies present in the system [12] , [23] , [32] , [33] . Our density functional theory results suggest an increase in the effective single-ion anisotropy of CrI 3 when brought in proximity to CrCl 3 . On the other hand, thanks to the induced ferromagnetic coupling, the CrCl 3 layer now sees an effective anisotropy field that depends both on the interfacial ferromagnetic coupling as well as the anisotropy of CrI 3 , which is expected to enlarge the spin-wave gaps for both the materials. This is consistent with the observed increase of T C for both 1L CrI 3 /FL CrCl 3 and 2L CrI 3 /FL CrCl 3 systems. Fig. 2: Temperature dependence of the magnetism of 2L CrI 3 and 2L CrI 3 /FL CrCl 3 heterostructure. MOKE signal in the 2L CrI 3 region ( a ) and the 2L CrI 3 /FL CrCl 3 heterostructure region ( b ) as a function of perpendicular magnetic field at different temperatures. Critical fields H 1 , H 1 * , H 2 * and magnitudes in the change of MOKE signal ∆ θ 1 , ∆ θ 1 * , ∆ θ 2 * of magnetic transitions are labeled. c Temperature dependence of the critical fields of magnetic transitions. PM paramagnetic. The critical fields are extracted from the peak of derivative d θ K /d H and the error bars are the peak widths. d Temperature dependence of the magnitudes in the change of MOKE signal at magnetic transitions. Solid curves are fitted by a power-law equation [11] . The critical temperatures T C and T C * are indicated. The error bars are the uncertainties in extracting the transition magnitudes. Full size image To better understand the observations, we explore the magnetic ground states of the CrI 3 /CrCl 3 bilayer using first-principles calculations (Supplementary Text 2 ). We find that the perpendicular ferromagnetic state (↑↑) is more favorable than three other magnetic configurations: perpendicular antiferromagnetic state (↑↓), the states that one layer is out-of-plane polarized while the other in-plane polarized (↑→ or →↑). Further consideration on magnetic dipole-dipole interaction and different commensurate twist angles (0° and 30°) does not undermine the favorable perpendicular ferromagnetic state. The interlayer exchange energy J inter in CrI 3 /CrCl 3 can be approximated by the energy difference between perpendicular antiferromagnetic and ferromagnetic configurations [17] . We estimate J inter ≈ −77 (−64) μJ/m 2 for 0° (30°)-twisted CrI 3 /CrCl 3 , compared to the reported interlayer exchange ~80 μJ/m 2 in 2L CrI 3 [32] , [34] , [35] . Such interfacial exchange coupling in the heterostructure wins over the in-plane anisotropy of CrCl 3 and results in the out-of-plane magnetic order in the CrCl 3 layer next to CrI 3 , in agreement with our observations. We next turn to explore the electrical tunability of the observed interfacial magnetism. A unique aspect of the CrI 3 /CrCl 3 heterostructure, when compared with previously explored monolayer and/or homobilayer systems [14] , [15] , [36] , is the absence of structural inversion symmetry. The Neumann’s principle [37] states that the spin-charge coupling is dictated by the symmetries of the system. We thus expect to observe spin-charge coupling phenomena for the interlayer magnetic order. In particular, breaking of structural inversion allows for direct electric-field modification of the magnetic anisotropy and the interlayer exchange interactions via terms of the form (see detailed discussions in Supplementary Text 3 ): 
    E_(m_i,σ_i)=(σ_1-σ_2)(β_1m_z1^2+β_2m_z2^2+β_3m_1·m_2),
 (1) where \({{{{{{\bf{m}}}}}}}_{i}\) , \({\sigma }_{i}\) are the magnetization and charges of the respective layers, \(({\sigma }_{1}-{\sigma }_{2})\sim\) electric field and \({\beta }_{{{{{\mathrm{1,2,3}}}}}}\) parameterizes the strength of respective interactions. Microscopically, the electric-field control of interfacial magnetic interactions could arise from electric-field-induced changes in the orbital occupancy in conjunction with spin-orbit interactions. Such a mechanism has attracted significant interest for constructing low-dissipation spintronic memory and logic devices [38] , [39] . To check the electric-field tuning of the observed interfacial magnetism, we fabricated a dual-gated 1L CrI 3 /FL CrCl 3 device, as shown in Fig. 3a, b . This structure allows us to study the magnetization of the CrI 3 /CrCl 3 heterostructure (as well as that of the 1L CrI 3 region in the same device) under the top-gate voltage V tg and back-gate voltage V bg . The two voltages are converted to electrostatic doping density n and displacement field D (Methods). 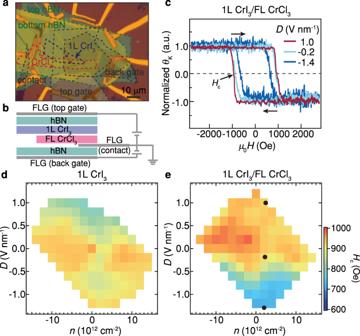Fig. 3: Electrical control of the magnetism in 1L CrI3/FL CrCl3heterostructure. a,bOptical micrograph and schematic structure of a dual-gated 1L CrI3/FL CrCl3device. Three few-layer graphene (FLG) flakes are used as back/top gates and the contact to the stack.cNormalized MOKE signal as a function of perpendicular magnetic field in 1L CrI3/FL CrCl3heterostructure under different displacement fieldsD= −1.4, −0.2, 1.0 V nm−1. Coercive fieldHcas a function of electrostatic doping densitynand displacement fieldDof 1L CrI3(d) and 1L CrI3/FL CrCl3heterostructure (e), respectively. The black dots inecorrespond to the MOKE curves inc. The data are taken at the spots marked by red ina. Figure 3c shows the coercive field ( H c ) in 1L CrI 3 /FL CrCl 3 heterostructure increases from ~700 Oe to ~1000 Oe when the D is tuned from −1.4 V nm −1 to 1 V nm −1 , indicating the enhancement of the magnetic anisotropy of the interfacial ferromagnetism in the heterostructure. The full mappings in Fig. 3d, e present the extracted H c as a function of both n and D in 1L CrI 3 and the 1L CrI 3 /FL CrCl 3 heterostructure, respectively. A quite weak modulation of H c is observed in 1L CrI 3 , suggesting that the magnetism of 1L CrI 3 can hardly be tuned under the range of gating voltages of this work. Separate experiments on FL CrCl 3 demonstrate that the magnetism of CrCl 3 also can hardly be tuned by electrostatic gating (Supplementary Fig. 5d ). However, significant tunability of the H c is observed by the D applied to the heterostructure. Such a dramatic tunability in the CrI 3 /CrCl 3 is in agreement with the electric field control of interfacial magnetic interactions allowed by the structural symmetry breaking, predicted in the above theoretical analysis. The intriguing electrical tunability allowed by symmetry breaking is also observed in a heterostructure containing a bilayer CrI 3 (Supplementary Text 4 ). Fig. 3: Electrical control of the magnetism in 1L CrI 3 /FL CrCl 3 heterostructure. a , b Optical micrograph and schematic structure of a dual-gated 1L CrI 3 /FL CrCl 3 device. Three few-layer graphene (FLG) flakes are used as back/top gates and the contact to the stack. c Normalized MOKE signal as a function of perpendicular magnetic field in 1L CrI 3 /FL CrCl 3 heterostructure under different displacement fields D = −1.4, −0.2, 1.0 V nm −1 . Coercive field H c as a function of electrostatic doping density n and displacement field D of 1L CrI 3 ( d ) and 1L CrI 3 /FL CrCl 3 heterostructure ( e ), respectively. The black dots in e correspond to the MOKE curves in c . The data are taken at the spots marked by red in a . Full size image In summary, we studied the interfacial magnetism in CrI 3 /CrCl 3 heterostructures and demonstrated the interfacial ferromagnetic coupling between neighboring CrI 3 and CrCl 3 layers. The demonstrated ability to engineer magnetoelectric phenomena by breaking symmetries via vdW heterostructures provides opportunities for vdW spintronics. The compatible hybrids of 2D magnets with other quantum materials, such as unconventional superconductors, ferroelectrics or topological materials are predicted to demonstrate exotic topological phases and many-body interactions [6] , [12] , [13] , as well as to design new spintronic devices and therefore are highly desirable for further study. Crystal growth Single crystal CrI 3 was synthesized using the chemical vapor transport (CVT) method [40] . The Cr powder and iodine pieces were mixed with a stoichiometric ratio and loaded into a quartz tube (inner diameter, 10 mm; length, 180 mm). The quartz tube was sealed under vacuum and then transferred to a double temperature zones furnace. The temperatures of the hot and cold ends of the furnace were set at 650 °C and 550 °C, respectively. The growth with such a temperature gradient lasted for 7 days. Finally, the furnace was shut down, and the quartz tube naturally cooled down to room temperature. The black plate-like CrI 3 crystals can be found at the cold end of the quartz tube. Single crystal CrCl 3 was grown by the CVT method. The commercial CrCl 3 polycrystal powder (99.9%) was sealed in a silica tube with a length of 200 mm and an inner diameter of 14 mm. The tube was pumped down to 0.01 Pa and sealed under vacuum, and then placed in a two-zone horizontal tube furnace. The two growth zones were raised slowly to 973 K and 823 K for 2 days, and then held there for another 7 days. After that, the furnace was shut down and cooled down naturally. Shiny, plate-like crystals with lateral dimensions of up to several millimeters can be obtained from the growth. Device fabrication FL CrI 3 , CrCl 3 and hexagonal boron nitride (hBN) flakes are exfoliated onto the silicon wafer covered by 285-nm thermal oxide layer. Flakes with proper thickness are selected by optical contrast [23] and later confirmed by AFM and MOKE measurements. CrI 3 flakes used in this work have 1~2 layers and the FL CrCl 3 flakes are around 5~10 nm (0.6 nm for each layer) thick. Heterostructures of CrI 3 and CrCl 3 are fabricated by the dry-transfer method and encapsulated between two hBN flakes with a typical thickness of ~10 nm. Specifically, a stamp made of a thin polycarbonate and polydimethylsiloxane is then employed to pick up the flakes in sequence under an optical microscope. In the end, the finished stack is deposited onto the target substrate with polycarbonate on top which is removed by chloroform afterwards. The whole process is performed inside a glovebox to avoid material degradation. The exposure time to air is kept below ten minutes before transferring the fabricated sample into the measurement chamber and pumping down. For the dual-gated heterostructure device and magnetic tunneling junction device, FL graphene flakes are exfoliated and integrated into the stack following the above processes. The target substrate is pre-patterned with electrodes fabricated by standard e-beam lithography, Au/Ti deposition and lift-off processes. The stack is carefully aligned and transferred onto the target pattern to make contact between graphene flakes and electrodes. MOKE microscopy The polarization of a linearly polarized light reflected from a magnetic material will be rotated by a Kerr angle θ K , which is proportional to the magnetization of the material. In this work, the incident light is normal to the sample plane and MOKE is in the polar geometry, meaning that the magnetic vector being probed is perpendicular to the sample surface and parallel to the incident light. A balanced photodetector and lock-in method are used to obtain the MOKE signal. A laser is used here with wavelength of 633 nm and power of 5 µW. The sample is placed in a helium-flow optical cryostat with the temperature down to 6 K and magnetic field (perpendicular to sample surface) up to 5 T. The laser is focused onto the sample surface by an objective with the spot diameter of 0.5 µm. Electrical control of the dual-gated device Top-gate and back-gate voltages can be applied to the FL graphene gates in the heterostructure device, while the graphene contact to the heterostructure is grounded. The dual-gate structure allows independent control of the doping density and displacement field applied on the heterostructure. The doping density n and displacement field D are extracted by the simple parallel plate capacitor model. For simplicity, the CrI 3 /CrCl 3 heterostructure is regarded as one channel, on which the doping density and electric field are applied. The quantum capacitance of CrI 3 and CrCl 3 is much larger than that of graphene due to the nearly flat bands of these two magnetic semiconductors [15] . Therefore, only geometric capacitances \({C}_{{{\mbox{bg}}}}\) and \({C}_{{{\mbox{tg}}}}\) are considered. The doping density and displacement field can be written as \(n={C}_{{{\mbox{bg}}}}\cdot {V}_{{{\mbox{bg}}}}+{C}_{{{\mbox{tg}}}}\cdot {V}_{{{\mbox{tg}}}}\) and \(D=({D}_{{{\mbox{bg}}}}+{D}_{{{\mbox{tg}}}})/2=({\varepsilon }_{{{\mbox{bg}}}}\cdot {V}_{{{\mbox{bg}}}}/{d}_{{{\mbox{bg}}}}-{\varepsilon }_{{{\mbox{tg}}}}\cdot {V}_{{{\mbox{tg}}}}/{d}_{{{\mbox{tg}}}})/2\) , respectively. The relative dielectric constant of hBN [14] is ε bg = ε tg = 3. For the device in Fig. 3 , the thicknesses of bottom hBN and top hBN are obtained by AFM measurement to be d bg = 19.6 nm and d tg = 14.9 nm, respectively.